Molecular determinants of selective clearance of protein inclusions by autophagy Protein quality control is essential for cellular survival. Failure to eliminate pathogenic proteins leads to their intracellular accumulation in the form of protein aggregates. Autophagy can recognize protein aggregates and degrade them in lysosomes. However, some aggregates escape the autophagic surveillance. Here we analyse the autophagic degradation of different types of aggregates of synphilin-1, a protein often found in pathogenic protein inclusions. We show that small synphilin-1 aggregates and large aggresomes are differentially targeted by constitutive and inducible autophagy. Furthermore, we identify a region in synphilin-1, necessary for its own basal and inducible aggrephagy and sufficient for the degradation of other pro-aggregating proteins. Although the presence of this peptide is sufficient for basal aggrephagy, inducible aggrephagy requires its ubiquitination, which diminishes protein mobility on the surface of the aggregate and favours the recruitment and assembly of the protein complexes required for autophagosome formation. Our study reveals different mechanisms for cells to cope with aggregate proteins via autophagy and supports the idea that autophagic susceptibility of prone-to-aggregate proteins may not depend on the nature of the aggregating proteins per se , but on their dynamic properties in the aggregate. Macroautophagy (henceforth referred to as autophagy) is a process that facilitates degradation of intracellular components through the sequestration of portions of the cytosol inside double-membrane vesicles that then fuse with lysosomes. This degradative mechanism has generated considerable interest because of its ability to eliminate proteins organized into aggregates (Agg) that are no longer amenable for degradation by other proteolytic systems. In fact, upregulation of autophagy has been shown to be beneficial in slowing down the progression of disease in animal models for different protein conformational disorders, including neurodegenerative diseases such as Huntington’s disease, amyotrophic lateral sclerosis and Parkinson’s disease [1] , [2] . The recognition of oligomeric insoluble cytosolic proteins by the autophagic machinery is still under study, but the participation of cargo-recognition molecules is now well-supported. Proteins such as p62 and NBR1 can simultaneously bind LC3, an essential component of the limiting membrane of the autophagosome, and different ubiquitin moieties displayed on the surface of the aggregated proteins to be degraded [3] , [4] , [5] . However, whether or not this is a universal mechanism of recognition or if all protein inclusions are susceptible to cellular removal by autophagy is still debatable. In fact, in yeast, two distinct types of intracellular protein Agg have been identified, based on their susceptibility to degradation by the proteasome [6] . These Agg also differ in their levels of ubiquitination and associated components. Mammalian equivalents of these two discrete types of Agg remain elusive. We have previously shown that autophagic clearance of aggresome (Agm)-like inclusions in mammals is a selective phenomenon influenced by the protein composition of the inclusion [7] . Activation of autophagy was enough to facilitate the removal of certain aggregation-prone protein inclusions, whereas this manipulation did not have an impact on the levels of other aggregated proteins. Failure to eliminate these proteins was not due to alterations in the autophagic process, as removal of other organelles and proteins occurred normally, but rather due to a failure to recruit the autophagic components to these Agg. Interestingly, when mixed inclusions were formed, the presence of the ‘autophagy-removable’ protein was enough to recruit the autophagic machinery and favour the removal of the protein. This observation highlights that certain properties of the proteins undergoing aggregation are required for recruiting the autophagic-lysosomal machinery to the Agm and facilitate its disposal by autophagy. In this study, we have investigated the factors that define amenability of Agm towards autophagic clearance using synphilin-1 (Sph1) as an example of ‘autophagy-removable’ protein. Sph1 has been detected in Lewy bodies (LBs) associated with different α-synucleinopathies such as Parkinson’s disease, diffuse Lewy body disease and multiple system atrophy [8] , [9] . Expression of Sph1 is also increased in the cortices of patients suffering from dementia with LB, Parkinson’s disease and the LB variant of Alzheimer’s disease [10] . Distinct regions of Sph1 define its ability to form either multiple small Agg or a single large perinuclear Agm [11] . The formation of small Agg of Sph1 is determined by the coiled-coil and ankyrin-like repeat domain 2 of Sph1 (termed ‘CC-ANK2’), whereas its translocation into Agm upon proteasome inhibition requires the presence of another N-terminally located ANK1 domain. We have used these protein variants to investigate whether Sph1 Agg and Agm exhibit similar susceptibility toward autophagy. We have found that clearance of Agg and Agm occurs via different types of autophagy. Although Agg are constitutively cleared by basal autophagy, Agm can only be removed by inducible autophagy. Furthermore, we have identified the specific region in Sph1 that is necessary and sufficient to mediate its autophagic removal when present both in Agg and Agm. Ubiquitination of this specific region modifies the dynamic properties of the proteins in the Agm and facilitates the assembly of initiators required for autophagosome formation directly on the surface of the Agm. By contrast, ubiquitination of the Sph1 motif is not required to promote Agg removal by basal autophagy. Our study suggests that manipulations aimed at mimicking these posttranslational modifications on the surface of autophagic-resistant protein inclusions could have therapeutic potential in some protein conformational disorders. Autophagy of Agm and Agg of Sph1 variants We have chosen Sph1 as a model protein to study autophagy of Agm-like inclusions because Sph1 Agm are readily removed by autophagy [7] ; co-aggregation of Sph1 with proteins that escape autophagic surveillance such as p38 (AIMP-2) promotes their autophagy [7] , and the contribution of the different regions of Sph1 to this aggregation have been well-characterized [11] . In fact, we confirmed that formation of Sph1 Agg upon proteasome inhibition in cells expressing different Sph1 deletion mutants is determined by the CC-ANK2 domain, whereas its organization into Ag requires the presence of the ANK1 domain ( Supplementary Fig. S1b shows that levels of the different Sph1 mutants were comparable after proteasome inhibition). To investigate possible differences in the autophagic susceptibility of Sph1 Agm and Agg, we compared the clearance of full-length (FL) Sph1 with three truncated variants, namely ACA, CACT and NA ( Fig. 1 ). Upon proteasome inhibition, FL and ACA Sph1 form both Agm and Agg, CACT Sph1 forms Agg, and NA Sph1 forms Agm ( Supplementary Fig. S1 ). To investigate the effect of basal and inducible (stimulated by starvation) autophagy, after proteasomal inhibition cells were maintained for 24 h in serum-supplemented (serum+) or serum-free medium (serum−) in the presence or absence of the autophagy inhibitor 3-methyladenine (3-MA), which permits tracking clearance independently of inclusion formation. 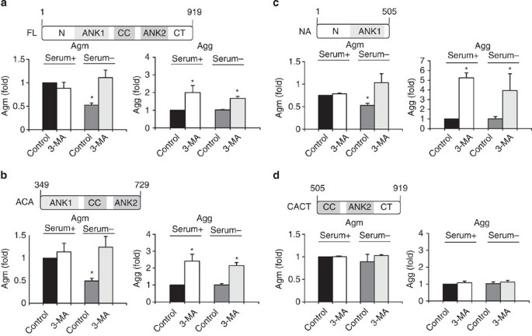Figure 1: Agm and Agg of truncated Sph1 variants exhibit different autophagic susceptibility. (a–d) Formation of protein inclusions in SY5Y cells expressing FL (a) or the indicated truncated forms of Sph1 (b–d) was induced by 12 h lactacystin treatment. After extensive washes, cells were maintained in serum-supplemented (serum+) or serum-free (serum−) media, and in the absence (Control) or presence of 10 mM 3-MA, an inhibitor of macroautophagy. Graphs show the relative fold difference in the number of cells containing either Sph1 Agm (left) or Agg (right) observed under different recovery conditions. Values are mean+s.e. (n=4). *Significant versus serum+ condition. See alsoSupplementary Figs S1–S5. Figure 1: Agm and Agg of truncated Sph1 variants exhibit different autophagic susceptibility. ( a – d ) Formation of protein inclusions in SY5Y cells expressing FL ( a ) or the indicated truncated forms of Sph1 ( b – d ) was induced by 12 h lactacystin treatment. After extensive washes, cells were maintained in serum-supplemented (serum+) or serum-free (serum−) media, and in the absence (Control) or presence of 10 mM 3-MA, an inhibitor of macroautophagy. Graphs show the relative fold difference in the number of cells containing either Sph1 Agm (left) or Agg (right) observed under different recovery conditions. Values are mean+s.e. ( n =4). *Significant versus serum+ condition. See also Supplementary Figs S1–S5 . Full size image As previously shown, induction of autophagy by starvation significantly reduced the number of cells containing FL Sph1 Agm, but this effect was prevented by 3-MA ( Fig. 1a ). Inhibition of autophagy did not affect Agm content in cells maintained in the presence of serum, supporting the inability of basal autophagy to clear FL Sph1 Agm ( Fig. 1a ). In contrast, blockage of basal autophagy increased (~2-fold) the number of FL Sph1 Agg-positive cells, but further induction of autophagy by starvation did not have any additional effect over basal clearance ( Fig. 1a ). Similar results were observed when considering number and percentage of cellular area occupied by FL Agg per cell, whereas the average size of the Agg remained unchanged ( Supplementary Fig. S2 ). Similar results were obtained for Agm and Agg of Sph1 containing only the central core region (ANK1-CC-ANK2, ACA Sph1; Fig. 1b and Supplementary Fig. S2 ). These results support that the amino and carboxy termini of Sph1 do not contribute to modulate Sph1 autophagic clearance. To separately analyse clearance of Sph1 Agm and Agg, we used the truncated variants lacking the CC-ANK2 domain (NA Sph1) or the ANK1 domain (CACT Sph1) that form preferentially only Agm or Agg, respectively ( Supplementary Fig. S1 ). The NA Sph1 Agm were amenable to inducible autophagy ( Fig. 1c ), whereas CACT Sph1 Agg were insensitive to both basal and inducible autophagy ( Fig. 1d and Supplementary Fig. S2 ). Analysis of the small population of cells containing Agm of CACT Sph1 revealed that these structures were no longer removed by basal or inducible autophagy ( Fig. 1d ). The viability of cells expressing the different Sph1 mutants was unaltered ( Supplementary Fig. S3 ). Interestingly, only the ANK1-containing Sph1 mutants accumulate in the insoluble pellet fractions upon autophagy inhibition with 3-MA treatment ( Supplementary Fig. S4 ), further confirming that the ANK1 domain in Sph1 is important for autophagy of both Sph1 Agm and Agg. As assembly of F-actin is required for basal autophagy but not for inducible autophagy [12] , we optimized treatment with latrunculin A, an actin polymerization inhibitor to disrupt the actin network without affecting Agm formation (that only occurs with prolonged (17 h) treatments ( Supplementary Fig. S5a ). Blockage of basal autophagy by the short latrunculin A treatment resulted in significant accumulation of Sph1 Agg (FL and ACA), similar to the one observed with 3-MA inhibition. However, elimination of the ANK1 domain (CACT Sph1 Agg) made these inclusions no longer amenable to basal autophagic clearance and, hence, insensitive to changes in this process ( Supplementary Fig. S5b ). Using embryonic fibroblasts from mice knock-out (KO) for the essential autophagy-related (Atg) gene Atg5 (Atg5 KO mouse embryonic fibroblast (MEF)), we confirmed that although the propensity of the Sph1 proteins to form Agm or Agg upon lactacystin treatment was the same as in wild-type (WT) MEFs ( Fig. 2a–c ), and levels of Agm (for FL, ACA and CACT Sph1) were comparable in both groups, they displayed marked accumulation of FL and ACA Agg already at basal conditions ( Fig. 2a–c ). In agreement with the findings in SY5Y cells, the number of CACT Sph1 Agg was not altered by the absence of functional autophagy ( Fig. 2c ), supporting that the loss of the ANK1 domain abolished their susceptibility to this removal. Similarly, starvation reduced FL and ACA Sph1 Agm in WT MEF, but did not have any effect in Atg5 KO MEF ( Fig. 2d–e ) or in the levels of Agm and Agg lacking the ANK1 domain ( Fig. 2f ). 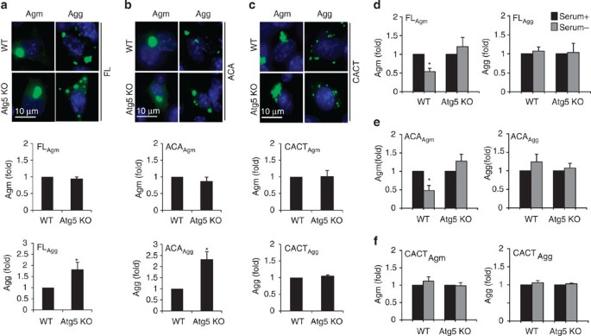Figure 2: Effect of genetic blockage of autophagy on clearance of Agm and Agg of Sph1 variants. (a–c) Top: fluorescence images of Agm and Agg observed in MEFs from WT and Atg5 KO mice expressing FL (a), or the indicated truncated Sph1 proteins (b–c) treated with lactacystin (12 h) and recovered in basal conditions (serum+). Graphs show the relative fold difference in the number of cells containing either Sph1 Agm (middle) or Agg (bottom). Values are mean+s.e. (n=3). *Significant versus control. (d–f) Relative fold difference in the number of FL (d) or truncated (e–f) Sph1 Agm (left) and Agg (right) in WT and Atg5 KO mice MEFs incubated in serum+ or serum− conditions. Values are mean+s.e. (n=3). *Significant versus serum+ condition. Figure 2: Effect of genetic blockage of autophagy on clearance of Agm and Agg of Sph1 variants. ( a – c ) Top: fluorescence images of Agm and Agg observed in MEFs from WT and Atg5 KO mice expressing FL ( a ), or the indicated truncated Sph1 proteins ( b – c ) treated with lactacystin (12 h) and recovered in basal conditions (serum+). Graphs show the relative fold difference in the number of cells containing either Sph1 Agm (middle) or Agg (bottom). Values are mean+s.e. ( n =3). *Significant versus control. ( d – f ) Relative fold difference in the number of FL ( d ) or truncated ( e – f ) Sph1 Agm (left) and Agg (right) in WT and Atg5 KO mice MEFs incubated in serum+ or serum− conditions. Values are mean+s.e. ( n =3). *Significant versus serum+ condition. Full size image Both chemical and genetic blockage of autophagy support that basal and inducible autophagy contribute differently to the removal of Agm and Agg, and highlight that the ANK1 domain in Sph1 contains the molecular determinants responsible for efficient autophagic removal of Sph1 protein inclusions. ANK1 domain in Sph1 promotes autophagic removal of p38 Agm Co-aggregation of Sph1 with p38 can promote the autophagic removal of p38 Agm, otherwise resistant to autophagy [7] . To identify the region(s) of Sph1 important to facilitate p38 removal, we co-expressed HA-p38 with the different Sph1 proteins. We found that most p38 (35–60%) associated with Sph1 proteins as Agm ( Fig. 3 ). Interestingly, even for CACT Sph1, which exists mainly as small Agg on its own ( Fig. 2c and Supplementary Fig. S1 ), the presence of p38 influenced it towards Agm formation ( Fig. 3d ), thus supporting that both proteins are able to influence each other’s aggregation properties. 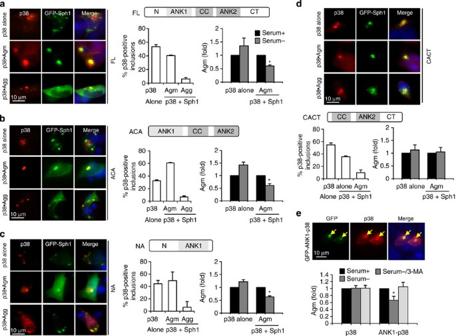Figure 3: The ANK1 domain in Sph1 proteins is required for autophagic removal of p38 Agm. (a–d) Left: fluorescence images of SY5Y cells co-expressing HA-p38 (red) and GFP (green) forms of FL (a) or the indicated truncated Sph1 (b–d). Cells were treated with lactacystin (12 h) and recovered in the presence or absence of serum. Graphs: percentage of p38 existing alone in Agm or co-aggregating with Sph1 in the forms of Agm or Agg (left), and susceptibility of p38 existing on its own in Agm or co-aggregating with Sph1 proteins in Agm toward serum-stimulated autophagic clearance (right). Values are expressed as folds Agm in the presence of serum and are mean+s.e. (n=3). *Significant versus serum+ condition calculated using Student’st-test. (e) Autophagic susceptibility of Agm formed by p38 and ANK1-p38 fusion proteins. Values are mean+s.e. (n=3). *Significant versus control group calculated using Bonferroni test. See alsoSupplementary Fig. S6. Figure 3: The ANK1 domain in Sph1 proteins is required for autophagic removal of p38 Agm. ( a – d ) Left: fluorescence images of SY5Y cells co-expressing HA-p38 (red) and GFP (green) forms of FL ( a ) or the indicated truncated Sph1 ( b – d ). Cells were treated with lactacystin (12 h) and recovered in the presence or absence of serum. Graphs: percentage of p38 existing alone in Agm or co-aggregating with Sph1 in the forms of Agm or Agg (left), and susceptibility of p38 existing on its own in Agm or co-aggregating with Sph1 proteins in Agm toward serum-stimulated autophagic clearance (right). Values are expressed as folds Agm in the presence of serum and are mean+s.e. ( n =3). *Significant versus serum+ condition calculated using Student’s t -test. ( e ) Autophagic susceptibility of Agm formed by p38 and ANK1-p38 fusion proteins. Values are mean+s.e. ( n =3). *Significant versus control group calculated using Bonferroni test. See also Supplementary Fig. S6 . Full size image Upon induction of autophagy, the number of Agm containing only p38 remained unchanged, as previously reported [7] . By contrast, Agm of p38 co-aggregated with FL, ACA or NA Sph1 showed significant reduction ( Fig. 3a–c ) that was no longer observed when p38 co-aggregated with Sph1 lacking the ANK1 domain (CACT; Fig. 3d ). Therefore, the ANK1 domain of Sph1 is required to target other protein inclusions for autophagic clearance. In fact, direct fusion of the ANK1 domain to the N terminus of GFP-p38 (hereafter referred to as ANK1-p38; Supplementary Fig. S6a ) significantly improved the susceptibility of p38 Agm towards starvation-induced autophagic clearance, except when autophagy was inhibited with 3-MA ( Fig. 3e ). This improved clearance was not due to global upregulation of cellular autophagy, but rather a specific effect mediated by ANK1 in the Agm ( Supplementary Fig. S6b ). Thus, both co-expression and fusion studies support that the ANK1 domain of Sph1 possesses the capacity to target ‘autophagic-resistant’ p38 Agm for degradation by macroautophagy. ANK1-dependent recruitment of autophagic machinery to Agm Inclusions that elude autophagic clearance fail to recruit key components of the autophagic-lysosomal machinery [7] . We examine whether the ANK1 domain contributes to the recruitment of this machinery and found that LAMP1 colocalized with ACA Sph1 Agm and Agg, which contain ANK1 domains ( Fig. 4a ), and that starvation increased LAMP1 association with Agm but not with Agg (in agreement with our clearance data Fig. 1b ). In both cases, lysosomal inhibition significantly increased the percentage of ACA Sph1 Agg co-stained with LAMP1, as expected from the removal of Agg by basal autophagy ( Fig. 4a ). In contrast, colocalization of LAMP1 with Agg of the Sph1 missing the ANK1 region (CACT) was minimal ( Fig. 4a ). Co-aggregation of p38 with all Sph1 proteins (FL, ACA and NA), except for CACT Sph1, or fusion of the ANK1 domain to p38 enhanced the recruitment of LAMP1 to p38-positive Agm ( Fig. 4b and Supplementary Fig. S7 ). 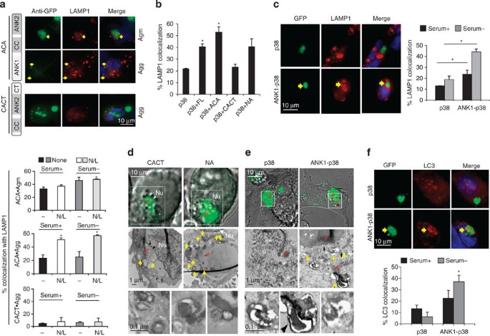Figure 4: ANK1 domain facilitates recruitment of autophagic-lysosomal compartments to Agm and Agg. (a) Top: colocalization of LAMP1 (red) with Agm and Agg of ACA and CACT Sph1 proteins highlighted by anti-GFP (green) in SY5Y cells. Arrows indicate colocalization. Bottom: percentage LAMP1 colocalization with Agm and Agg in cells maintained in serum+ or serum− media, treated or not with lysosomal inhibitors (N/L). (b) Percentage LAMP1 colocalization with Agm in cells co-expressing HA-p38 and the indicated Sph1 proteins maintained in the absence of serum. (c) Left: colocalization of LAMP1 (red) with GFP-p38 and -ANK1-p38 Agm in SY5Y cells maintained in the absence of serum. Arrows indicate colocalization. Right: percentage LAMP1 colocalization with p38 and ANK1-p38 Agm in cells maintained in the presence or absence of serum. (d,e) Correlative light and electron microscopy of SY5Y cells expressing the indicated GFP-tagged Sph1 truncations (d), or p38 and ANK1-p38 (e). Top: phase-contrast fluorescence microscopy; middle: electron micrographs of the boxed region; bottom: higher magnification examples of autophagic vacuoles (yellow arrows).#Location of the Agm or Agg structures in both the fluorescence images and the corresponding micrographs. (f) Top: colocalization of LC3 (red) with GFP-p38 and -ANK1-p38 Agm in SY5Y cells maintained in the absence of serum. Arrows indicate colocalization. Bottom: percentage colocalization of LC3 with the fluorescent proteins. Values in all graphs represent mean+s.e. (n=3). *Significant versus serum+ condition (a,c,f) or p38 Agm (b) calculated using Bonferroni test. See alsoSupplementary Fig. S7. Figure 4: ANK1 domain facilitates recruitment of autophagic-lysosomal compartments to Agm and Agg. ( a ) Top: colocalization of LAMP1 (red) with Agm and Agg of ACA and CACT Sph1 proteins highlighted by anti-GFP (green) in SY5Y cells. Arrows indicate colocalization. Bottom: percentage LAMP1 colocalization with Agm and Agg in cells maintained in serum+ or serum− media, treated or not with lysosomal inhibitors (N/L). ( b ) Percentage LAMP1 colocalization with Agm in cells co-expressing HA-p38 and the indicated Sph1 proteins maintained in the absence of serum. ( c ) Left: colocalization of LAMP1 (red) with GFP-p38 and -ANK1-p38 Agm in SY5Y cells maintained in the absence of serum. Arrows indicate colocalization. Right: percentage LAMP1 colocalization with p38 and ANK1-p38 Agm in cells maintained in the presence or absence of serum. ( d , e ) Correlative light and electron microscopy of SY5Y cells expressing the indicated GFP-tagged Sph1 truncations ( d ), or p38 and ANK1-p38 ( e ). Top: phase-contrast fluorescence microscopy; middle: electron micrographs of the boxed region; bottom: higher magnification examples of autophagic vacuoles (yellow arrows). # Location of the Agm or Agg structures in both the fluorescence images and the corresponding micrographs. ( f ) Top: colocalization of LC3 (red) with GFP-p38 and -ANK1-p38 Agm in SY5Y cells maintained in the absence of serum. Arrows indicate colocalization. Bottom: percentage colocalization of LC3 with the fluorescent proteins. Values in all graphs represent mean+s.e. ( n =3). *Significant versus serum+ condition ( a , c , f ) or p38 Agm ( b ) calculated using Bonferroni test. See also Supplementary Fig. S7 . Full size image Using correlative light and fluorescence electron microscopy [13] that allows simultaneous visualization of the green fluorescent protein (GFP) inclusions and the surrounding region at the ultrastructural level, we found that structures morphologically compatible with autophagic vacuoles were more abundant around NA Sph1 Agm ( Fig. 4d ) and ANK1-p38 Agm ( Fig. 4e ), when compared with Agg formed by CACT Sph1, which lacks the ANK1 domain and p38 Agm, respectively. Immunofluorescence (IF) against the autophagic marker LC3 confirmed the autophagic nature of these vesicles and demonstrated significantly higher colocalization with ANK1-p38 Agm compared with p38 Agm ( Fig. 4f ). Therefore, the ANK1 domain augments the autophagic susceptibility of Agm and Agg by mediating efficient recruitment of the autophagic-lysosomal machinery. ANK1-mediated aggrephagy is independent of p62 and NBR1 To understand how ANK1 facilitates recruitment of the autophagic-lysosomal machinery to p38 Agm, we first characterized the interactions of the cargo-recognition proteins p62 and NBR1 with the different p38 inclusions. As seen previously, p62 was detectable by IF in both autophagy-sensitive (Sph1 and ANK1-p38) and -insensitive (p38) Agm ( Fig. 5a ). We then photobleached Agm formed in cells expressing mCherry-p62 alone or in conjunction with Sph1 or the p38 variants, and analysed the recovery kinetics of mCherry-p62 fluorescence in these Agm. In all Agm, less than 20% of the initial mCherry-p62 fluorescence was recovered after photobleaching, supporting that a large fraction of p62 molecules did not exchange with non-bleached surrounding molecules ( Fig. 5b and Supplementary Fig. S8 ). We found that p62 exists in all Agm as two populations with different mobility (diffusible and immobile) and that co-aggregation with other proteins increases the p62 diffusible fraction but reduces its mobility (longer t 1/2 recovery time). However, similar percentage of mobile p62 and p62 recovery time were found in Agm containing Sph1 or the different p38 variants ( Fig. 5b and Supplementary Fig. S8 ), supporting that the presence of ANK1 did not alter p62 kinetics in the p38 Agm. 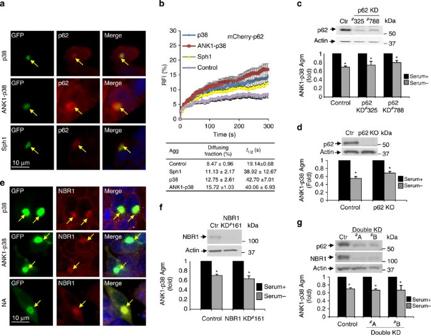Figure 5: Cargo-recognition proteins p62 and NBR1 are not required for autophagic clearance of ANK1-p38. (a) Fluorescence images showing colocalization patterns of the indicated GFP-p38 variants and Sph1 (green) with endogenous p62 (red) in SY5Y cells. Arrows indicate colocalization. (b) Quantitative FRAP analysis of mCherry-p62 expressed alone (control) or co-expressed with the indicated GFP-Sph1 and -p38 variants. Top: time course of changes in relative fluorescence intensity (RFI); bottom: percentage of p62 in the diffusing fraction and diffusion time (t1/2). Values are mean+s.e. of ten cells analysed over three different experiments. Representative images are shown inSupplementary Fig. S8. (c–d) Top: IBs for p62 and actin in control and p62 knockdown (p62 KD#325 or#788) SY5Y cells (c); and in control and p62 KO MEFs (d). Bottom: autophagic clearance of GFP-ANK1-p38 Agm in the same cells in response to serum removal. (e) Fluorescence images of GFP-p38, -ANK1-p38 and -NA Sph1 Agm in SY5Y cells immunostained for endogenous NBR1. Arrows indicate colocalization. (f,g) Top: IBs for NBR1, p62 and actin in control and NBR1 knockdown (NBR1 KD#161) SY5Y cells (f), and in control and p62/NBR1 double knockdown (Double KD#A or#B) SY5Y cells (g). Bottom: autophagic clearance of GFP-ANK1-p38 Agm in the same cells. For all densitometric analyses, values are mean+s.e. (n=3). *Significant versus serum+ condition. See alsoSupplementary Fig. S8–S11. Figure 5: Cargo-recognition proteins p62 and NBR1 are not required for autophagic clearance of ANK1-p38. ( a ) Fluorescence images showing colocalization patterns of the indicated GFP-p38 variants and Sph1 (green) with endogenous p62 (red) in SY5Y cells. Arrows indicate colocalization. ( b ) Quantitative FRAP analysis of mCherry-p62 expressed alone (control) or co-expressed with the indicated GFP-Sph1 and -p38 variants. Top: time course of changes in relative fluorescence intensity (RFI); bottom: percentage of p62 in the diffusing fraction and diffusion time ( t 1/2 ). Values are mean+s.e. of ten cells analysed over three different experiments. Representative images are shown in Supplementary Fig. S8 . ( c – d ) Top: IBs for p62 and actin in control and p62 knockdown (p62 KD # 325 or # 788) SY5Y cells ( c ); and in control and p62 KO MEFs ( d ). Bottom: autophagic clearance of GFP-ANK1-p38 Agm in the same cells in response to serum removal. ( e ) Fluorescence images of GFP-p38, -ANK1-p38 and -NA Sph1 Agm in SY5Y cells immunostained for endogenous NBR1. Arrows indicate colocalization. ( f , g ) Top: IBs for NBR1, p62 and actin in control and NBR1 knockdown (NBR1 KD # 161) SY5Y cells ( f ), and in control and p62/NBR1 double knockdown (Double KD # A or # B) SY5Y cells ( g ). Bottom: autophagic clearance of GFP-ANK1-p38 Agm in the same cells. For all densitometric analyses, values are mean+s.e. ( n =3). *Significant versus serum+ condition. See also Supplementary Fig. S8–S11 . Full size image We then analysed the effect of knocking down ( Fig. 5c ) or knocking out p62 (p62 KO MEF; Fig. 5d ) on Agm kinetics and found that reduction of p62 levels did not significantly affect formation of Agm or global autophagic activity ( Supplementary Fig. S9 ). Significant clearance of the ANK1-p38 Agm upon induction of autophagy still occurred in both p62-defective cells ( Fig. 5c ), and clearance of ANK1-containing Sph1 Agg and Agm was unperturbed ( Supplementary Figs S10–S11 ). Consequently, changes in the ability to recruit p62 or in p62 dynamics in both Agm and Agg are not behind the enhanced autophagic susceptibility provided by ANK1. Similarly, we did not find differences in the ability of p38 and ANK1-containing Agm to recruit NBR1 ( Fig. 5e ), and ablation of NBR1 or of both NBR1 and p62 did not prevent the removal of ANK1-p38 Agm or of Agm and Agg of the ANK1-containing Sph1 proteins ( Fig. 5f and Supplementary Figs S9d,e and S10 ). These results suggest that the ANK1-mediated autophagic clearance of both Agm and Agg is not dependent on p62 or NBR1 proteins. ANK1 enhances recruitment of the autophagy-initiation complex Despite p62 and NBR1 being detected both in p38 and ANK1-p38 Agm, in the absence of the ANK1 region LC3 failed to be recruited to the p38 Agm ( Fig. 4f ). We next examined whether the presence of ANK1 could help recruitment of the initiators of autophagy upstream of LC3 [14] directly to the Agm. Immunostaining for key components of the autophagy nucleation complex [15] , [16] , [17] revealed the presence of beclin-1 in both p38- and ANK1-containing Agm, whereas Vps34 and Atg14L were only associated in the form of a ‘rim’ with the ANK1-containing Agm ( Fig. 6 and Table 1 ). These findings support that the ANK1 region may facilitate the assembly of the phosphoinositide-3-kinase nucleation complex directly on the surface of Agm. We observed that higher percentage of ANK1-containing Agm were ‘coated’ with DFCP-1, a downstream effector of the nucleation complex in phagophore formation [18] , [19] , when compared with p38 Agm ( Fig. 6d ). We propose ANK1 may facilitate recruitment of LC3 to the Agm by facilitating the assembly of autophagy-initiation complexes on the surface of the Agm ( Table 1 ). 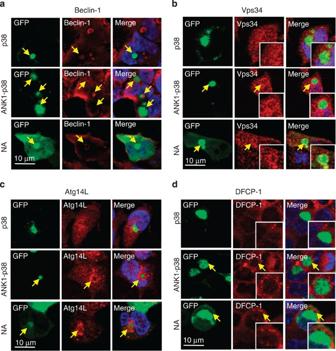Figure 6: Preferential assembly of autophagosome nucleating complexes in ANK1-containing Agm. (a–d) Fluorescence images of GFP-p38, -ANK1-p38 and -NA Sph1 Agm in SY5Y cells immunostained for endogenous beclin-1 (a), Vps34 (b), Atg14L (c) and DFCP-1 (d). Arrows indicate colocalization. Figure 6: Preferential assembly of autophagosome nucleating complexes in ANK1-containing Agm. ( a – d ) Fluorescence images of GFP-p38, -ANK1-p38 and -NA Sph1 Agm in SY5Y cells immunostained for endogenous beclin-1 ( a ), Vps34 ( b ), Atg14L ( c ) and DFCP-1 ( d ). Arrows indicate colocalization. Full size image Table 1 Association of different Atg proteins with the indicated aggresome types. Full size table Intrinsic properties of Agm determine their autophagy We attempted to demonstrate a direct interaction between the ANK1 region and specific components of the autophagy nucleation complex. However, immunoprecipitation of ANK1 from the soluble cellular fraction did not bring along any of the autophagic proteins observed in the Agm (data not shown), suggesting that the association of autophagy nucleation proteins with ANK1 only occurs when ANK1-containing proteins are already organized into the Agm. If that is the case, it is possible that distinctive characteristics of these Agm may facilitate assembly of the autophagy nucleation proteins directly on their surface, but not on those lacking the ANK1 region. We compared the biophysical properties of p38 with and without ANK1 in Agm using fluorescent recovery after photobleaching (FRAP) analysis and found a significant reduction in the fraction of diffusible p38 in the Agm when bearing the ANK1 domain ( Fig. 7a ), in agreement with their more compact appearance by electron microscopy ( Fig. 4e ). 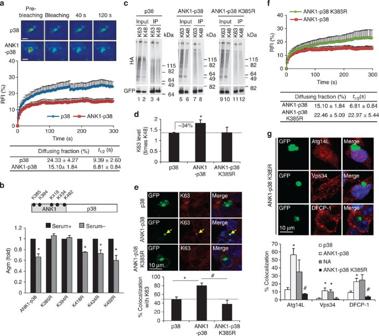Figure 7: ANK1-mediated ubiquitination reduces Agm protein mobility and favours Atg recruitment. (a) Quantitative FRAP analysis of the indicated GFP-p38 variants. Top: representative images. Middle: time course of changes in relative fluorescence intensity (RFI). Bottom: percentage of proteins in the diffusing fraction and diffusion time (t1/2). Values are mean+s.e. of ten cells analysed over three different experiments. Scale bars, 10 μm (b) Top: schematic showing all lysine (K) residues in ANK1 domain of Sph1 that may serve as potential ubiquitination site(s). Bottom: relative fold difference in the number of Agm formed by WT and the different ‘K to R’ mutants of ANK1-p38 fusion protein in SY5Y cells maintained in the presence or absence of serum. (c) IBs for HA (top) and GFP (bottom) of total lysates (Input) and GFP immunoprecipitates (IP) from the cell lysates of SY5Y cells co-transfected with the indicated HA–ubiquitin constructs and GFP-p38 or -ANK1-p38 WT or mutant K385R in the presence of lactacystin. (d) Quantification of the levels of each p38 protein ubiquitinated via K63 compared with K48 ubiquitination. Values were corrected by levels of GFP immunoprecipitated. (e) Top: IF for GFP and K63-linked ubiquitin (red) of SY5Y cells expressing GFP-p38 or -ANK1-p38 WT and mutant K385R (green). Arrows indicate colocalization. Bottom: percentage of Agm positive for K63-linked ubiquitin. (f) Quantitative FRAP analysis of GFP-ANK1-p38 K385R and GFP-ANK1-p38 as in (a). Values are mean+s.e. of ten cells analysed over three different experiments. (g) Top: representative images of GFP-ANK1-p38 K385R Agm in SY5Y cells immunostained for Atg14L, Vps34 and DFCP-1. Bottom: percentage of p38 variant and NA Sph1 Agm that colocalized with Atg14L, Vps34 and DFCP-1 under serum− conditions. Values in all graphs represent mean+s.e. (n=3). *Significant versus serum+ condition or p38 Agm.#Significant versus ANK1-p38 Agm. Significance calculated using Bonferroni test. See alsoSupplementary Fig. S8. Figure 7: ANK1-mediated ubiquitination reduces Agm protein mobility and favours Atg recruitment. ( a ) Quantitative FRAP analysis of the indicated GFP-p38 variants. Top: representative images. Middle: time course of changes in relative fluorescence intensity (RFI). Bottom: percentage of proteins in the diffusing fraction and diffusion time ( t 1/2 ). Values are mean+s.e. of ten cells analysed over three different experiments. Scale bars, 10 μm ( b ) Top: schematic showing all lysine (K) residues in ANK1 domain of Sph1 that may serve as potential ubiquitination site(s). Bottom: relative fold difference in the number of Agm formed by WT and the different ‘K to R’ mutants of ANK1-p38 fusion protein in SY5Y cells maintained in the presence or absence of serum. ( c ) IBs for HA (top) and GFP (bottom) of total lysates (Input) and GFP immunoprecipitates (IP) from the cell lysates of SY5Y cells co-transfected with the indicated HA–ubiquitin constructs and GFP-p38 or -ANK1-p38 WT or mutant K385R in the presence of lactacystin. ( d ) Quantification of the levels of each p38 protein ubiquitinated via K63 compared with K48 ubiquitination. Values were corrected by levels of GFP immunoprecipitated. ( e ) Top: IF for GFP and K63-linked ubiquitin (red) of SY5Y cells expressing GFP-p38 or -ANK1-p38 WT and mutant K385R (green). Arrows indicate colocalization. Bottom: percentage of Agm positive for K63-linked ubiquitin. ( f ) Quantitative FRAP analysis of GFP-ANK1-p38 K385R and GFP-ANK1-p38 as in ( a ). Values are mean+s.e. of ten cells analysed over three different experiments. ( g ) Top: representative images of GFP-ANK1-p38 K385R Agm in SY5Y cells immunostained for Atg14L, Vps34 and DFCP-1. Bottom: percentage of p38 variant and NA Sph1 Agm that colocalized with Atg14L, Vps34 and DFCP-1 under serum− conditions. Values in all graphs represent mean+s.e. ( n =3). *Significant versus serum+ condition or p38 Agm. # Significant versus ANK1-p38 Agm. Significance calculated using Bonferroni test. See also Supplementary Fig. S8 . Full size image We then set to elucidate how the ANK1 region influenced mobility of aggregating proteins in Agm to facilitate their autophagic removal. We postulated that ANK1-dependent changes may not be related to its amino acid sequence per se —as this sequence is not conserved in other aggregate-prone proteins degraded by autophagy, but that it could serve as a platform for posttranslational modifications that help in stabilizing the protein in Agm, and thus permit efficient assembly of the autophagy nucleation complex on their surface. Given that the N-terminal region of Sph1 (including its ANK1 domain) is ubiquitinated by multiple E3 ubiquitin ligases [20] , a modification already linked to aggrephagy [6] , [21] , we mutated all the five lysine residues located within the ANK1 region to arginine and found that elimination of K385 and K394 abolished the autophagic clearance of ANK1-p38 ( Fig. 7b ). These results confirm the importance of ubiquitination in mediating ANK1-dependent autophagy but were, to some extent, surprising because p38 has been shown to be already ubiquitinated in protein inclusions [7] , [22] . Consequently, we compared next the type of ubiquitin linkage in p38 and ANK1-p38, looking in particular for K63 ubiquitination previously linked to aggrephagy [21] . Analysis of the ubiquitin profiles of p38 immunoprecipitated from cells co-expressing HA-K63 and -K48 ubiquitin mutants (that only form K63 and K48 ubiquitination, respectively), showed that although both linkages occur in all the p38 variants ( Fig. 7c ), there were quantitative differences; although p38 and mutant ANK1-p38 K385R displayed almost equal K48 and K63 ubiquitination, ANK1-p38 showed preference for K63 ubiquitination ( Fig. 7d ). IF with an antibody for K63-linked ubiquitin confirmed that ~80% of ANK1-p38 Agm were positive for K63-linked ubiquitin, whereas only 44 and 38% of p38 and mutant ANK1-p38 K385R Agm, respectively, were co-stained with K63-linked ubiquitin ( Fig. 7e ). These results support that presence of ANK1 favours K63 over K48 ubiquitination on p38. FRAP experiments on mutant ANK1-p38 K385R Agm revealed that the ANK1-induced decrease in protein mobility was dependent on the capability of ANK1 to become ubiquitinated, because the decrease in the diffusible fraction was no longer observed in mutant ANK1-p38 K385R Agm ( Fig. 7f ). In fact, although the addition of the K385R-mutated ANK1 region slows down the exchange of p38 between the Agm and the surrounding region (longer recovery time), it is not enough to reduce the fraction of mobile protein, which is only attained when ubiquitination of ANK1 remains intact ( Fig. 7f ). FRAP analysis of lysosomes stained with LysoTracker in close proximity to Agm of p38 and Sph1 variants did not reveal differences in their mobility discarding global changes in the viscosity of that region ( Supplementary Fig. S12 ). IF analysis revealed a significant decrease in association of Atg14L, Vps34 and DFCP-1 with the K385R-mutated ANK1 Agm ( Fig. 7g ), further confirming that changes in protein mobility at the surface of the Agm are responsible for the differences in the association of autophagy-related proteins to these structures. To investigate the importance of ANK1 K63 ubiquitination in Agg removal, we created the same K385R and K394R mutations in FL Sph1 protein, capable of generating both Agm and Agg. Although both mutations abolished clearance of FL Sph1 Agm by starvation-induced autophagy, like in the case of ANK1-p38 ( Fig. 8a ), they did not affect basal autophagic degradation of the corresponding Agg ( Fig. 8b ). In fact, IF shows that only Agm but not Agg were preferentially K63 ubiquitinated ( Fig. 8c ). These results indicate that K63 ubiquitination is required for Agm removal by inducible autophagy, but not for degradation of Agg by basal quality-control autophagy. 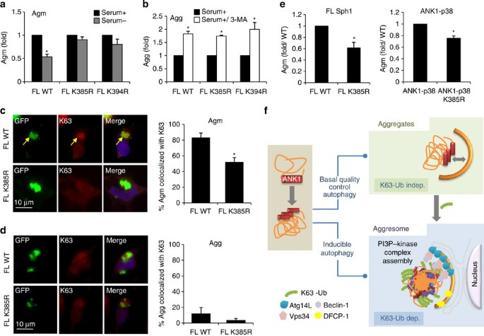Figure 8: ANK1-mediated ubiquitination is dispensable for basal autophagy of Sph1 Agg. (a,b) Autophagic clearance of Agm (a) or Agg (b) formed by FL WT and mutant K385R or K394R GFP-Sph1 in SY5Y cells, in response to serum removal (a) or upon blockage of basal autophagy with 3-MA (b). (c,d) Left: Agm (c) or Agg (d) of FL GFP-Sph1 (green) immunostained for endogenous K63-linked ubiquitin (red) in SY5Y cells. Arrows in (c) indicate colocalization. Right: percentage of Agm (c) or Agg (d) positive for K63-linked ubiquitin. (e) Formation of WT and mutant K385R FL Sph1 (left) and ANK1-p38 (right) Agm in response to proteasome inhibition. Values in all graphs represent mean+s.e. (n=3). *Significant versus serum+ condition (a,b) or WT FL Sph1 or ANK1-p38 (c–e). (f) Schematic model of the contribution of the ANK1 region and K63 linkage of this region to removal of Agg and Agms through different types of autophagy. Figure 8: ANK1-mediated ubiquitination is dispensable for basal autophagy of Sph1 Agg. ( a , b ) Autophagic clearance of Agm ( a ) or Agg ( b ) formed by FL WT and mutant K385R or K394R GFP-Sph1 in SY5Y cells, in response to serum removal ( a ) or upon blockage of basal autophagy with 3-MA ( b ). ( c , d ) Left: Agm ( c ) or Agg ( d ) of FL GFP-Sph1 (green) immunostained for endogenous K63-linked ubiquitin (red) in SY5Y cells. Arrows in ( c ) indicate colocalization. Right: percentage of Agm ( c ) or Agg ( d ) positive for K63-linked ubiquitin. ( e ) Formation of WT and mutant K385R FL Sph1 (left) and ANK1-p38 (right) Agm in response to proteasome inhibition. Values in all graphs represent mean+s.e. ( n =3). *Significant versus serum+ condition ( a , b ) or WT FL Sph1 or ANK1-p38 ( c – e ). ( f ) Schematic model of the contribution of the ANK1 region and K63 linkage of this region to removal of Agg and Agms through different types of autophagy. Full size image Lastly, as we have previously shown that K63 ubiquitination has dual role of promoting Agm formation and autophagic targeting [23] , we analysed whether K63 ubiquitination is behind the previously described role of ANK1 in Agm formation [11] . When we compared the levels of Agm formed during the period of proteasome inhibition by WT FL Sph1 or WT ANK1-p38 with their corresponding K385R mutant variants, we observed a significant reduction in the number of Agm for the K385R mutants of both proteins ( Fig. 8e ). These findings support that K63 ubiquitination of ANK1 drives formation of autophagy-competent Agm during proteasomal malfunction for disposal by inducible autophagy, as this is likely a more efficient way of eliminating these aggregated proteins than constitutive autophagy of small aggregates. In summary, our studies support the existence of different mechanisms for cells to cope with aggregate proteins via autophagy. Although basal autophagy constitutively degrades small Agg, K63 ubiquitination of aggregated proteins is utilized to generate Agm amenable for removal by inducible autophagy. The presence of K63 ubiquitination makes Agm competent for autophagy by reducing the mobility of the aggregating protein in these structures, and favouring, thus, in situ assembling of the autophagic-initiating machinery. In this study, we have found that the degradation of protein inclusions by autophagy is influenced by their aggregation properties and have identified distinctive functions of basal and inducible autophagy in the clearance of protein inclusions. Whereas small Agg are mainly removed by basal quality-control autophagy, cells use inducible autophagy to dispose of proteins organized into large perinuclear Agm ( Fig. 8f ). Using Sph1 as a model protein, we have identified that its ANK1 domain is necessary and sufficient for autophagic clearance of both Agg by basal autophagy and Agm by inducible autophagy. ANK1-mediated autophagic clearance of Agm depends on its ability to undergo K63 ubiquitination, which in turn reduces the mobility of the aggregating protein in Agm. The compactness of the Agm does not influence the binding of cargo-recognition molecules, but instead determines the ability to assemble the autophagy-initiation machinery on the surface of the Agm. By contrast, K63 ubiquitination is dispensable in ANK1-mediated clearance of Agg by basal quality-control autophagy. In fact, K63 ubiquitination in the ANK1 of these Agg favours their progression into autophagy-amenable Agm, which could be a safety mechanism when their cellular load overcomes basal autophagy ( Fig. 8f ). Although multiple monoubiquitination and K63 ubiquitination have been implicated in aggregation events, only Agm enriched in K63 ubiquitination are preferentially removed by autophagy [4] , [21] , [24] . Our analysis supports the hypothesis that subtle changes in the relative proportion of different ubiquitin linkages in Agm, rather than a complete switch in the type of linkage, are sufficient to modify their autophagic amenability. This is consistent with the fact that tissues from autophagy-deficient mice accumulate a variety of ubiquitin linkages rather than a specific type [25] . It is possible that different types of ubiquitin moieties in Agm fulfil very different functions that could include seeding, assistance on self-assembly, binding of cargo-recognition molecules and, as shown in this study, the locking of the aggregate proteins into compact structures to facilitate the assembly of the autophagy-initiation complexes on their surface. Formation and priming through K63 ubiquitination of Agm for disposal by autophagy appears to be an inducible phenomenon that is more relevant during cellular stress, such as proteasome inhibition. Interestingly, protein mobility and ubiquitination status also have a role in defining the degradation of distinct protein aggregates in yeast [6] . In contrast to yeast, in which aggregating compartments with different removal susceptibility localize in different cellular regions and contain or lack ubiquitin, both autophagy-insensitive and -sensitive Agms in mammalian cells are localized perinuclearly and are always ubiquitinated, albeit differently [6] , [7] , [21] . Different efficiency in basal quality-control autophagy between mammals and yeast maybe behind the differences in the need for distinct protein aggregation subcompartments. Basal and inducible autophagy processes are differently regulated and involve distinctive molecular components. In this study, we provide evidence of differences in the cargo targeted by each of these types of autophagy. The same protein is removed by basal autophagy when in small aggregates and by inducible autophagy once sequestered into Agms. Interestingly, ANK1 is important for both types of aggrephagy, but ANK1-mediated basal aggrephagy, contrary to induced aggrephagy, is independent of K63 ubiquitination. The presence of regions amenable to K63 linkage such as ANK1 may determine the switch between basal and inducible aggrephagy. ANK1-mediated basal and inducible autophagy are independent of the cargo-recognition proteins p62 and NBR1. Recent studies support that more than one type of cargo-recognition molecules exist for facilitating the removal of same kinds of autophagic substrates and that they can function independently, or in conjunction in process like mitophagy [26] , [27] , [28] , [29] , [30] and selective bacterial autophagy [31] , [32] , [33] . We consider unlikely that ANK1 acts by enhancing cooperation between p62 and NBR1, as depletion of both simultaneously did not affect clearance of ANK1-containing Agm and Agg, but cannot discard that ANK1 may bring to Agm yet-to-be-identified cargo-recognition molecules. Our dissection of the arrival of mammalian Atg proteins to Agm supports that the lower levels of LC3 detected in p38 Agm are likely a consequence of the observed inability of these Agm to recruit Atg14L and Vps34. The ANK-independent presence of beclin-1 in Agm in absence of the other components of the kinase complex may be due to their entrapment in Agm. It is also possible that additional functional molecules of beclin-1 arrive at the ANK1-containing Agm along with Atg14L and Vps34. The interaction of nucleation Atgs with Agm observed in our study may be different from other conditions in which these proteins have been described to become inactive as they get trapped in protein inclusions [34] , as we found efficient recruitment of downstream molecules such as DFCP-1. The fact that both Vps34 and Atg14L, and in many instances K63 linkages, adopt a distinctive ‘rim’ distribution in the periphery of the ANK1-p38 Agm, as well as the lower mobility observed in the surface of these Agm compared with p38 Agm, led us to hypothesize that the additional K63 linkages supplied by ANK1 lock the molecules of p38 at the Agm surface to provide a more stable platform for assembly of the autophagosome-initiation complex. These changes in the biophysical properties of the aggregating molecules could be facilitated by the more open and extended topology of the K63 linkages when compared with K48 linkages. The multiple functions of K63 ubiquitin chains in a single Agm could explain why they could become limiting in the autophagic clearance of Agm. The K63-linked ubiquitin normally detected in p38 are clearly sufficient for the formation of the Agm and for binding of the cargo-recognition proteins, p62 and NBR1, but insufficient for stabilizing p38 in the Agm. The ‘rim’ shape of K63-linked ubiquitin in the Agm supports that in addition to the amount, its distribution may also be important for this stabilizing and pro-Atg assembly function of K63-linked ubiquitin. Our results support the idea that autophagic susceptibility of prone-to-aggregate proteins may not depend on the nature of the aggregating protein per se , but on their dynamic properties once in the Agm. From an applied point of view, it should be, thus, possible to promote selective autophagic clearance of otherwise unmovable protein inclusions, through interventions (that is, small molecules) aimed at stabilizing the aggregating protein in the inclusion. Cell culture and transfections The neuroblastoma cell line SY5Y was from American Type Culture Collection. MEFs from Atg5 and p62 KO mice and their respective paired WT MEFs were gifts from Drs Noboru Mizushima (Tokyo Medical and Dental University, Japan) and Masaaki Komatsu (Tokyo Metropolitan Institute of Medical Science). All cells were cultured in DMEM medium (Sigma) in the presence of 10% fetal bovine serum. SY5Y cells and MEFs were transfected with the various expression vectors using Lipofectamine 2000 reagent (Invitrogen) according to the manufacturer’s instructions. Chemicals Sources of chemicals and antibodies were as previously described [7] . Antibodies were used for immunoblot (IB) and IF at the following concentrations: anti-LC3 (Cell Signaling Technology), 1:1,000 IB and 1:200 IF; anti-LAMP1 (Developmental Studies Hybridoma Bank), 1:3,000 IB and 1:300 IF; anti-GFP (Santa Cruz), 1:200 IF; anti-NBR1 (Abnova) 1:5,000 IB and 1:200 IF; anti-beclin-1 (Novus Biologicals), 1:200 IF; anti-Vps34 (Invitrogen), 1:100 IF; anti-K63-linked ubiquitin (Millipore), 1:500 IB and 1:100 IF; anti-actin (Abcam), 1:10,000 IB; anti-p62 (Enzo Life Sciences), 1:3,000 IB and 1:200 IF; anti-Atg14L (MBL), 1:100 IF; anti-DFCP-1 (Sigma), 1:100 IF; anti-p38 (Proteintech), 1:1,000 IB and 1:200 IF; anti-HA (Sigma), 1:3,000 IB and 1:200 IF; anti-GFP (Roche), 1:3,000 IB; and Alexa-labelled secondary antibodies (Invitrogen) and other fluorescent-labelled secondary antibodies (Jackson ImmunoResearch Laboratories) were all used at 1:5,000 IB and 1:500 IF. Plasmids construction Human p38 ( AIMP-2 ) gene was amplified from HA-p38 plasmid via PCR using forward primer 5′-TGC GCG TCG ACC ATG CCG ATG TAC CAG GTA-3′ and reverse primer 5′-CGC GGA TCC TGT AAA AAA GGA GCC AGG TT-3′, which incorporated 5′ Sal 1 and 3′ Bam H1 restriction sites to the p38 gene. The Sal 1/ Bam H1-restricted p38 PCR product was subcloned into pEGFP-N1 vector (Clontech Laboratories, Mountain View, CA, USA) to create the GFP-p38 construct. The ANK1 domain was amplified from FL GFP-Sph1 plasmid via PCR using forward primer 5′-CCG CTC GAG ATG AAT GGA AAC AAT CTA-3′ and reverse primer 5′-CAT GGT CGA CGC GCA CAG GGT GTG-3′ that incorporated 5′ Xho 1 and 3′ Sal 1 restriction sites to the ANK1 domain. The Xho 1/ Sal 1-restricted ANK1 domain was subsequently subcloned in frame to the N terminal of the p38 gene in GFP-p38 plasmid to create the GFP-ANK1-p38 fusion construct. Inclusion formation and autophagic clearance The susceptibility of various inclusions formed upon proteasomal inhibition toward autophagic removal was analysed as described [7] . Briefly, cells transfected with the protein of choice were first treated with 5 μM lactacystin for 12 h, and then washed and maintained for 24 h in serum-containing media (for basal autophagy) or serum-deprived media (for inducible autophagy) either in the presence or absence of the autophagy inhibitor, 10 mM 3-MA (Sigma). Cells were then fixed and analysed by IF for scoring as Agm- or Agg-containing cells according to the description in Supplementary Fig. S1c . Protein knockdown RNA interference of p62 and NBR1 expression in SY5Y cells was carried out using lentivirus carrying the respective short hairpin RNAs (shRNAs) as described [35] , [36] . Lentiviral transfer vectors containing shRNAs against p62 (NM_003900.2-325s1c1; NM_003900.2-788s1c1) and NBR1 (NM_031858.1-1620s1c1) from MISSION shRNA (Sigma) were separately co-transfected with the third-generation packaging constructs pMDLg/pRRE and pRSV-REV, and the G glycoprotein of VSV (pMD2.G) into HEK293T cells as envelop via calcium phosphate method. Lentiviral particles recovered from the culture media were used to transduce 2 × 10 5 SY5Y cells for 72 h. Thereafter, the cells were collected to check efficiency of knockdown by immunoblotting for the protein levels. Stable knockdown clones were created using puromycin selection. Site-directed mutagenesis The lysine to arginine (K–R) mutations in the ANK1 domain were introduced via PCR using the following mutagenic primers: K385R: forward 5′-CGCAACACTGAGAGGTTGACTCCAGC-3′ and reverse 5′-GCTGGAGTCACCTCTCAGTGTTGCG-3′; K394R: forward 5′-GCCTGGCCATTAGGAATGGTCAGTTG-3′ and reverse 5′-CAACTGACCATTCCTAATGGCCAGGC-3′; K418R: forward 5′-CTGAGTTGTTCTAGGGATTTTCCAAGC-3′ and reverse 5′-GCTTGGAAAATCCCTAGAACAACTCAG-3′; K434R: forward 5′-ATGGCCAGG AAAGGATTCTTCTGTG-3′ and reverse 5′-CACAGAAGAATCCTTTCCTGGCCAT-3′; K492R: forward 5′-GCTGGGGAAAGGCCCTCCCAG-3′ and reverse 5′-CTGGGAGGGCCTTTCCCCAGC-3′. GFP-ANK1-p38 and FL GFP-Sph1 plasmids were used as templates for the mutagenesis PCR. The resultant mutations were confirmed by sequencing. Immunocytochemistry and fluorescence microscopy Cells grown on coverslips were fixed with 3% formaldehyde, permeabilized with 0.1% Triton X-100 and stained for fluorescence microscopy as described previously. Lysosome staining was carried out by incubating cells with 100 nM LysoTracker for 30 min at 37 °C followed by three washes in PBS. Mounting medium contained DAPI (4′,6-diamidino-2-phenylindole) to highlight the cellular nucleus. Images were acquired with Axiovert 200 fluorescence microscope equipped with X63 objective or X100 objective, and 1.4 numerical aperture, subjected to deconvolution with the manufacturer’s software and prepared using Adobe Photoshop 6.0 software (Adobe Systems Inc., Mountain View, CA, USA). The number of aggregates per cell profile, the average size of the aggregates and the percentage cellular area occupied by the aggregates were analysed using the ‘analyse particles’ function in ImageJ software (NIH). The analysis was done on images with maximum projection of all Z-stack sections and thresholded with size (pixel 2 ) settings from 0.1 to 10, and circularity 0–1. A minimum of 20 cells per slide were quantified. Live cell imaging and photobleaching SY5Y cells expressing GFP-tagged p38, ANK1-p38, ANK1-p38 K385R and mCherry-p62, separately or in combination, were cultured on glass bottom 35 mm culture dishes (MatTek). Cells were maintained in minimum essential medium without phenol red, supplemented with 10% fetal bovine serum, sodium bicarbonate and HEPES buffer at 37 °C for the duration of the FRAP analysis using either the 488- or 543-nm laser wavelength for GFP and mCherry constructs, respectively. The recovery of fluorescence in the region of interest was monitored by capturing images every 3 s at a low power of laser in a time-course sequence. Average Agm-associated fluorescence intensity was determined using Leica Confocal software and the relative fluorescence intensity was calculated as the average of at least three data points. FRAP data were fit using Sigma Plot Software to two-phase exponential method. Correlative light and electron microscopy SY5Y cells expressing GFP-NA Sph1, -CACT Sph1, -p38 and -ANK1-p38 grown on grid glass bottom, 35-mm culture dish were recovered in serum-free medium for 6 h after proteasome inhibition. Vinblastine (5 μM) was added for the last 2 h of starvation to enhance the presence of autophagosomes. Thereafter, the cells were fixed, and confocal stacks as well as differential interference contrast images of transfected cells were acquired. Cells were then embedded in Epon and sectioned for electron microscopy analysis. The imaged cell was relocated in the block face and sectioned through. Sections were contrasted with lead citrate and uranyl acetate and serial sections of the cell of interest were documented at X10,000, X15,000 and X30,000 magnifications on a Hitachi 7,000 electron microscope. Confocal, differential interference contrast and transmission electron microscopic images were realigned and oriented using nuclear and other morphological landmarks. IB and immunoprecipitation Cells were lysed in cold RIPA lysis buffer and protein was quantified by the Lowry method, using BSA as a standard. After SDS–PAGE and immunoblotting, the proteins recognized by the specific antibodies were visualized by chemiluminescence methods (Western lightning ECL plus, PerkinElmer) and the membranes subjected to densitometric analysis using the ImageJ software (NIH). For immunoprecipitation, cells were lysed in RIPA lysis buffer containing 6 M urea with brief sonication, and the solubilized fraction was incubated with the corresponding primary antibodies overnight and with protein A/G beads (Amersham Biosciences) for 1 h. After washing, the immunoprecipitates were subjected to SDS–PAGE and immunoblotting. Statistical analysis Results are shown as mean±s.e. Statistical significance of the differences between groups was analysed using Student’s t -test unless otherwise stated. Difference were considered significant for P <0.05. How to cite this article: Wong, E. et al . Molecular determinants of selective clearance of protein inclusions by autophagy. Nat. Commun. 3:1240 doi: 10.1038/ncomms2244 (2012).